Hydrochromic conjugated polymers for human sweat pore mapping Hydrochromic materials have been actively investigated in the context of humidity sensing and measuring water contents in organic solvents. Here we report a sensor system that undergoes a brilliant blue-to-red colour transition as well as ‘Turn-On’ fluorescence upon exposure to water. Introduction of a hygroscopic element into a supramolecularly assembled polydiacetylene results in a hydrochromic conjugated polymer that is rapidly responsive (<20 μs), spin-coatable and inkjet-compatible. Importantly, the hydrochromic sensor is found to be suitable for mapping human sweat pores. The exceedingly small quantities (sub-nanolitre) of water secreted from sweat pores are sufficient to promote an instantaneous colorimetric transition of the polymer. As a result, the sensor can be used to construct a precise map of active sweat pores on fingertips. The sensor technology, developed in this study, has the potential of serving as new method for fingerprint analysis and for the clinical diagnosis of malfunctioning sweat pores. Materials that undergo colour changes in response to physical (heat, light, pressure, current and so on) and chemical/biochemical (solvent, pH, ligand–receptor interactions and so on) inputs serve as the key components in a number of sensor, display, switch and memory devices [1] , [2] , [3] , [4] , [5] , [6] . Among stimulus-responsive colorimetric substances investigated thus far, conjugated polymers [7] have gained special attention owing to their unique optical properties associated with the presence of extensively delocalized π-electron networks. As localized stimulation of conjugated polymers brings about changes in absorption and emission characteristics, these materials have been effectively utilized as sensor matrices [8] , [9] , [10] , [11] , [12] , [13] , [14] , [15] , [16] , [17] . Polydiacetylenes (PDAs) [18] , [19] , [20] , [21] , [22] , [23] , [24] , [25] , [26] , [27] , [28] possess unique structural features that differ from those of other conjugated polymers. As they are prepared by polymerization of self-assembled diacetylene monomers ( Fig. 1 ), PDAs are intrinsically supramolecular aggregates in which dense packing restricts conformational mobility of main chain backbones and enables extensive and efficient p-orbital overlap. As a result, PDAs generally have an absorption maximum at around 650 nm that corresponds to a blue colour. When the aggregated, blue-coloured supramolecular PDAs completely dissociate into individual PDAs upon exposure to an appropriate solvent, their side chains are able to rotate freely and, as a result, a blue-to-yellow colour transition occurs [29] , [30] . However, because of the presence of strong interchain interactions, PDAs are typically insoluble in common organic solvents. Instead, dissolution of unpolymerized residual diacetylene monomers and partially polymerized oligomers in common organic solvents creates voids in the PDA supramolecules, which leads to partial distortion of the polymer backbone and a blue-to-red (or purple) colour change [31] , [32] . 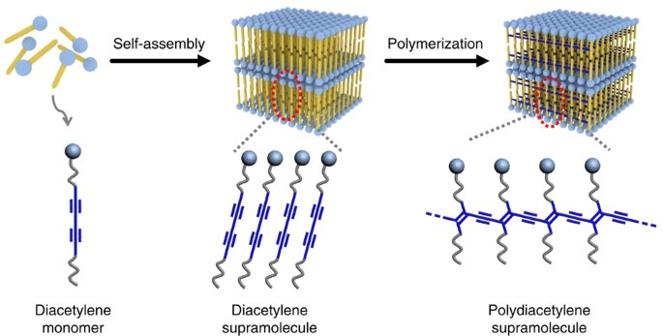Figure 1: Supramolecular polydiacetylene. Schematic for formation of a supramolecular PDA from a self-assembled diacetylene entity. Figure 1: Supramolecular polydiacetylene. Schematic for formation of a supramolecular PDA from a self-assembled diacetylene entity. Full size image We recently introduced conceptually new strategies, such as a protective layer approach [33] and a combinatorial method [34] , for the design of solvatochromic PDA sensor systems. Our continuing efforts in this area led to development of a new PDA, which contains hygroscopic elements in its headgroup and, consequently, is colorimetrically responsive to water. The hydrochromic PDA was found to undergo a dramatic and rapid structural change in the presence of water that brings about a blue-to-red colour transition. The new solvatochromic sensor system developed in this study possesses several significant features. First, although many solvatochromic PDA sensor systems that respond to organic solvents have been described [29] , [30] , [31] , [32] , [33] , [34] , a colorimetric PDA, which is responsive to pure water, has not yet been developed. Second, the hydrochromic PDA developed in this study is spin-coatable and inkjet-compatible, two important advantages when compared with conventional small molecule-based water-responsive sensors. Third, the colorimetric response of the sensor can be readily controlled by manipulation of the chain length of the diacetylene monomer and the hygroscopic element. This is a significantly meritorious property of PDAs that is not shared by other conjugated polymers and small molecule sensors. Fourth, the blue-to-red colorimetric transition is accompanied by the generation of red fluorescence, a feature that enables the PDA to serve as a ‘Turn-On’ functioning sensor. Last, the fluorescence ‘Turn-On’ PDA system is applicable to mapping human sweat pores. The results show that the very small amounts (<nanolitre) of water secreted from sweat pores are sufficient to promote an instantaneous blue-to-red colorimetric transition as well as a fluorescence ‘Turn-On’ of the polymer film, a phenomenon that enables precise mapping of active sweat pores on a human fingertip. Thus, the sensor technology developed in this study has the potential of serving as a new method for fingerprint analysis and for the clinical diagnosis of malfunctioning sweat pores. We believe that the observations made in the investigation will serve as the foundation for new applications of hydrochromic materials, beyond simply humidity sensing [35] and measurement of water contents in organic solvents [36] . The details of the investigation leading to these conclusions are described below. Discovery of the hydrochromic PDA The investigation described below was guided by the hypothesis that introduction of hygroscopic moieties into head groups of PDAs would lead to conjugated polymers that undergo significant water-promoted electronic changes. In order to explore this proposal, PDAs containing cesium carboxylate head groups were selected as potential targets owing to the typically highly hygroscopic nature of these ion complexes and the fact that the polymers can be readily prepared from commercially available diacetylene monomers. For example, a transparent gel is generated when an equimolar mixture of 10,12-pentacosadiynoic acid (PCDA, CH 3 (CH 2 ) 11 C≡C–C≡C(CH 2 ) 8 COOH) and cesium hydroxide in aqueous tetrahydrofuran (THF) is stirred for 1 h at an ambient temperature ( Supplementary Fig. 1a ). Inspection of a scanning electron microscope (SEM) image shows that the PCDA-Cs gel comprises thin-plate morphologies ( Supplementary Fig. 1b ) and a thin film is readily formed when the viscous gel is spin-coated on a solid substrate. UV irradiation (254 nm, 1 mW cm −2 , 30 s) of the coated film results in the formation of blue-coloured poly(PCDA-Cs; Fig. 2a ). 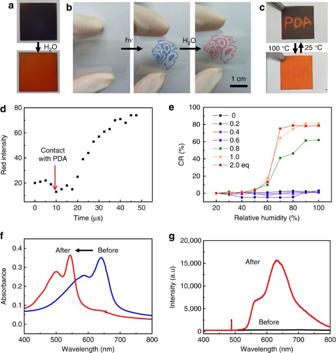Figure 2: Hydrochromic PDA. (a) Colorimetric transition of a poly(PCDA-CS) coated (thickness:ca.3.8 μm) PET film upon exposure to water. (b) Photographs of printed image of a PET film using a PCDA-Cs ink solution immediately following printing (transparent image), after UV irradiation (254 nm, 1 mW cm−2) for 30 s (blue-coloured image) and after exposure to water (red-coloured image). (c) A handwritten image of ‘PDA’ on a poly(PCDA-Cs)-coated PET film with a water-filled ballpoint pen at 25 °C (PDA image) and at 100 °C (PDA image disappears). (d) Time-dependent red intensity variations of a poly(PCDA-Cs) film during exposure to a water droplet. (e) Colorimetric response (CR) of a poly(PCDA-Cs) film as a function of molar equivalent of Cs ion to PCDA. The CR is calculated by using the well-known equation51CR=(PB0−PBf)/PB0× 100%, where PB0and PBfare the percent blue before and after the colour transition and PB=A640nm/[A640nm+A550nm]. (f,g) Water induced visible absorption (f) and emission (g) (excitation at 488 nm) spectral changes of a poly(PCDA-Cs) film upon hydration. Figure 2: Hydrochromic PDA. ( a ) Colorimetric transition of a poly(PCDA-CS) coated (thickness: ca. 3.8 μm) PET film upon exposure to water. ( b ) Photographs of printed image of a PET film using a PCDA-Cs ink solution immediately following printing (transparent image), after UV irradiation (254 nm, 1 mW cm −2 ) for 30 s (blue-coloured image) and after exposure to water (red-coloured image). ( c ) A handwritten image of ‘PDA’ on a poly(PCDA-Cs)-coated PET film with a water-filled ballpoint pen at 25 °C (PDA image) and at 100 °C (PDA image disappears). ( d ) Time-dependent red intensity variations of a poly(PCDA-Cs) film during exposure to a water droplet. ( e ) Colorimetric response (CR) of a poly(PCDA-Cs) film as a function of molar equivalent of Cs ion to PCDA. The CR is calculated by using the well-known equation [51] CR=(PB 0 −PB f )/PB 0 × 100%, where PB 0 and PB f are the percent blue before and after the colour transition and PB=A 640nm /[A 640nm +A 550nm ]. ( f , g ) Water induced visible absorption ( f ) and emission ( g ) (excitation at 488 nm) spectral changes of a poly(PCDA-Cs) film upon hydration. Full size image Interestingly, an immediate blue-to-red colorimetric response occurs when the poly(PCDA-Cs) film is exposed to a soft blow of human expiration ( Fig. 2a ; Supplementary Movie 1 ). The water-promoted colour change was found to occur even at low temperatures ( Supplementary Movie 2 ). In addition, the poly(PCDA-Cs) can be generated in an inkjet-compatible manner ( Fig. 2b , Supplementary Movie 3 ). To demonstrate this feature, a cartridge of a conventional thermal inkjet office printer was filled with an aqueous suspension of PCDA-Cs and then employed to print an image on a polyethylene terephthalate (PET) film (see Methods for details). Since monomeric PCDA-Cs does not absorb visible light, the printed image is not visible. However, UV irradiation with a hand-held laboratory 254 nm UV lamp for 10 s results in the formation of a blue-patterned image associated with formation of poly(PCDA-Cs). The image undergoes an instant blue-to-red colour change upon exposure to water. The versatility of the hydrochromic PDA-coated PET film was further demonstrated by utilizing it to create images with a ballpoint pen filled with water ( Fig. 2c ). Interestingly, the handwritten, red image disappears when the film is heated to 100 °C and reappears upon cooling the film to room temperature ( Supplementary Movie 4 ). This colour-switching phenomenon is likely a consequence of the fact that the poly(PCDA-Cs) film displays a reversible thermochromism ( Supplementary Fig. 2 ) and that the hydrochromism process is irreversible. The thermally controlled, reversible on-off image process can be repeated many times (>100) without losing the quality of the image. Probing the nature of the hydrochromism The rate of the water-promoted colorimetric response of the poly(PCDA-Cs) film was evaluated by employing a high-speed camera. The plot of intensity of the red colour as a function of time following exposure to a water droplet displayed in Fig. 2d demonstrates that a significant colour change occurs within 20 μs after water contacts the film and reaches a maximum after 40 μs. In order for the PDA to display effective hydrochromism, the molar equivalents of cesium ion in the PCDA complex needs to be greater than 0.8 ( Fig. 2e ). This observation suggests that a large portion of the PDA supramolecules needs to be in hygroscopic forms in order for an efficient colour change to occur. The hydrochromic behaviour of the poly(PCDA-Cs)-coated PET film was also probed by using visible absorption spectroscopy ( Fig. 2f ). Inspection of the spectra shows that a significant shift in the wavelength maximum from 640 to 540 nm takes place when the film is treated with water. In addition, because the blue-phase poly(PCDA-Cs) is nonfluorescent while its red-phase counterpart fluoresces, the water-promoted transition was also observed using emission spectroscopy ( Fig. 2g ). Analysis of the emission spectra shows that a fluorescence emission band centred at 630 nm (excitation: 488 nm) arises when the blue poly(PCDA-Cs) film is exposed to water. Finally, the results of Raman spectroscopic studies ( Supplementary Fig. 3 ) demonstrate that water causes shifts in the alkyne–alkene bands (2,079 and 1,452 cm −1 ) associated with poly(PCDA-Cs) to higher frequencies (2,120 and 1,515 cm −1 ), an observation that confirms that a typical [37] blue-to-red phase transition of PDA occurs in response to water. Important observations, which contribute to an understanding of the origin of the hydrochromic behaviour of the PDAs, were made in SEM and X-ray diffraction (XRD) studies. The SEM image shows that a morphological transition from strips to isolated aggregates takes place upon exposure of the poly(PCDA-Cs) film to water ( Fig. 3a ). The water-promoted morphological change of the film is also reflected in the results of XRD studies ( Fig. 3b ). Specifically, the initial blue-coloured PDA-Cs film comprises lamellar structures with an interlamellar distance of 4.81 nm, calculated by utilizing the Bragg’s law. Upon hydration, a new structure with an interlamellar distance of 6.19 nm is formed. The water-promoted increase in interchain distance should lead to partial distortion of the arrayed p-orbitals that is responsible for the blue-to-red colour change of the polymer ( Fig. 3c ). 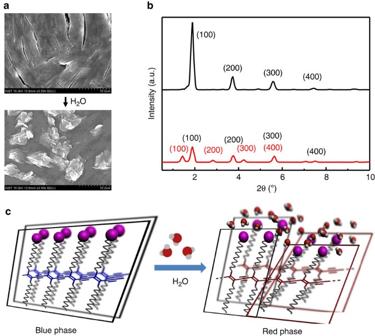Figure 3: Water-promoted morphological change. (a) SEM images of a poly(PCDA-Cs) film that displays a drastic morphological change upon hydration. (b) XRD spectra of a poly(PCDA-Cs) film before (black line) and after (red line) exposure to water. An interlamellar distance of 4.81 nm obtained before exposure to water and a new structure generated after exposure to water are indexed following the Bragg’s law. (c) Schematic representation of the water-promoted blue-to-red phase transformation of PDA supramolecules. The purple-coloured balls represent hygroscopic elements. Figure 3: Water-promoted morphological change. ( a ) SEM images of a poly(PCDA-Cs) film that displays a drastic morphological change upon hydration. ( b ) XRD spectra of a poly(PCDA-Cs) film before (black line) and after (red line) exposure to water. An interlamellar distance of 4.81 nm obtained before exposure to water and a new structure generated after exposure to water are indexed following the Bragg’s law. ( c ) Schematic representation of the water-promoted blue-to-red phase transformation of PDA supramolecules. The purple-coloured balls represent hygroscopic elements. Full size image Studies of complexes of PCDA that contain other metal cations indicate that films that comprises lithium, sodium and potassium salts of the polymer do not undergo the water-promoted colour transition while the film containing the poly(PCDA-Rb) complex forms a red colour upon being hydrated ( Supplementary Fig. 4 ). The results of contact angle measurements show that the hydrochromism of the polymer film is governed by the size of the counter cation in the PDA complex ( Supplementary Fig. 5 ). One meritorious feature of PDAs, which is not shared by other conjugated polymers, is associated with the fact that their colorimetric responses can be readily controlled by manipulation of the chain length of the diacetylene monomer and the head groups. In general, PDAs derived from diacetylenes with shorter alkyl chains are more sensitive to environmental stimulations than are those derived from longer alkyl chain monomers [38] . We have demonstrated that this phenomenon is also observed in the hydrochromism behaviour of PDAs. For example, as pointed out above no colorimetric transition takes place when the PDA derived from PCDA-K is exposed to water ( Supplementary Fig. 4 ). However, the PDA derived from 10,12-tricosadiynoic acid (TCDA)-K (two carbons shorter than PCDA) displays a blue-to-red colour transition initiated under 100% relative humidity (RH) conditions ( Fig. 4 ). In addition, poly(HCDA-K) obtained from HCDA, which contains a two carbon shorter chain than does TCDA, is even more sensitive to water in that its colour change takes place under RH 90% conditions. As summarized in Fig. 4 , proper combinations of diacetylene monomers and cations enable fabrication of hydrochromic PDA films that are responsive to specific levels of humidity. 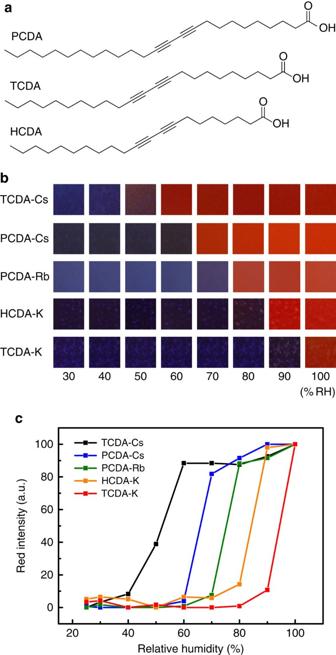Figure 4: Tuning of hydrochromic response. (a) Chemical structures of diacetylenic lipids: PCDA, TCDA, HCDA (8,10-heneicosadiynoic acid). (b) Colorimetric response of PDA films derived from various combinations of diacetylene monomers and ions under different humidity conditions. (c) Red intensity of the hydrochromic PDA films shown inbas a function of relative humidity. It is evident from the figures that colorimetric response of PDA films can be manipulated by choosing proper diacetylene monomers and cations. Figure 4: Tuning of hydrochromic response. ( a ) Chemical structures of diacetylenic lipids: PCDA, TCDA, HCDA (8,10-heneicosadiynoic acid). ( b ) Colorimetric response of PDA films derived from various combinations of diacetylene monomers and ions under different humidity conditions. ( c ) Red intensity of the hydrochromic PDA films shown in b as a function of relative humidity. It is evident from the figures that colorimetric response of PDA films can be manipulated by choosing proper diacetylene monomers and cations. Full size image Hydrochromic mapping of human sweat pores Every individual has discernably unique ridge patterns on their fingertips. Owing to the presence of sweat components (fatty acids, amino acids, inorganic salts and so on), these patterns are transferred to solid substrates when fingers touch the surface. Analyses of the fingerprint patterns left on solid surfaces have been unarguably one of the most convincing tools for the proof of an individual’s presence at a specific location and, as a result, a variety of techniques [39] , [40] , [41] , [42] , [43] , [44] , [45] , [46] have been developed for imaging and comparing these patterns. Close inspection of fingertips reveals that they contain permanent, immutable and unique pores that are distributed on the ridges. The possible use of pore analysis for personal identification was demonstrated by Locard [47] in studies that show that 20–40 pores are sufficient to generate patterns that are required for a human’s identity. When a finger touches a porous substrate, such as paper, nonvolatile sweat components from the fingertip become immobilized on the porous substrate, which because of its highly networked structure, limits free migration of the sweat components. As a result, dot images of the pores rather than complete ridge patterns that correspond to fingertip patterns become deposited on the substrate. Unfortunately, these pore dot images have been for the most part neglected owing to the fact that rapid, reliable and affordable fingertip pore mapping technologies have not been developed. Although modern high-resolution sensor systems (>1,000 d.p.i.) can be utilized to image fingertip pore patterns, they require complicated software, often contain false information owing to the presence of complicated ridge and pore structures and are incapable of distinguishing sweat-secreting active pores from those that are not functioning [48] . In light of the importance of pore mapping technologies, the water-promoted colour transition of the PDA-Cs film described above has great potential. In particular, if the blue-to-red transforming hydrochromic PDA were to be sufficiently sensitive to the small amounts of water present in sweat secreted from fingertips, it would be ideal for mapping sweat pores. In order to test this possibility, a fingerprint was deposited on the surface of a blue PDA-Cs film. Surprisingly, the polymer film became red instantaneously upon contact with the fingertip ( Fig. 5a ). Inspection of the contact area using an optical microscope showed that the image comprises many red-coloured dots ( Fig. 5b ). Fluorescence microscope analysis provided a clear image of the fingerprint in the form of emitting dots ( Fig. 5c ; Supplementary Movie 5 ). Raman spectroscopy was also employed to demonstrate that the typical structural transition of the PDA has occurred in the red microdot regions ( Fig. 5d ) [37] . 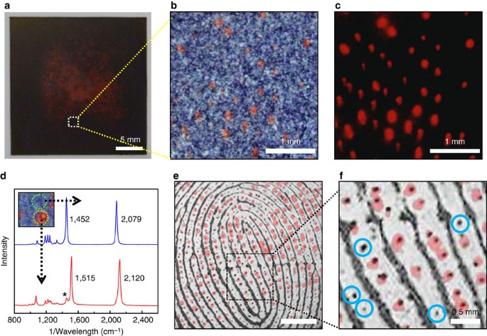Figure 5: Sweat pore mapping. (a) Photograph of a fingerprint image printed on a poly(PCDA-Cs) film (thickness:ca.3.8 μm). (b,c) Optical (b) and fluorescence (c) microscope images of the magnified fingerprint area marked ina. The fluorescence image was obtained with excitation at 510–550 nm. (d) Raman spectra of a poly(PCDA-Cs) film after fingerprinting. The small peak marked with * corresponds to the unconverted blue-phase PDA. (e) Superimposed image of contrast-enhanced fluorescence dots on a scanned fingerprint image. (f) Magnified image of the marked area ine. The dots inside the blue circles are pores that do not secret sweat. Figure 5: Sweat pore mapping. ( a ) Photograph of a fingerprint image printed on a poly(PCDA-Cs) film (thickness: ca. 3.8 μm). ( b , c ) Optical ( b ) and fluorescence ( c ) microscope images of the magnified fingerprint area marked in a . The fluorescence image was obtained with excitation at 510–550 nm. ( d ) Raman spectra of a poly(PCDA-Cs) film after fingerprinting. The small peak marked with * corresponds to the unconverted blue-phase PDA. ( e ) Superimposed image of contrast-enhanced fluorescence dots on a scanned fingerprint image. ( f ) Magnified image of the marked area in e . The dots inside the blue circles are pores that do not secret sweat. Full size image In order to gain more information about the origin of the microdots, the fluorescence patterns corresponding to the red dots were superimposed on a digitally scanned fingertip image ( Fig. 5e ). Inspection of the superimposed images ( Fig. 5e,f ) showed that the red-coloured microdots are located on the ridges of the fingertip. In addition, black-coloured microdots seen in the images are pores on fingertip ridges, most of which match with red dots that correspond to active sweat pores. Specifically, the dots inside the blue circles in Fig. 5f correspond to pores that do not secret sweat. These observations clearly demonstrate that the red dots are generated by PDA colour transitions promoted by water secreted from sweat pores. The reproducibility of the hydrochromic method for pore mapping was demonstrated by using superimpositions of three independently deposited fingerprints ( Fig. 6 ). 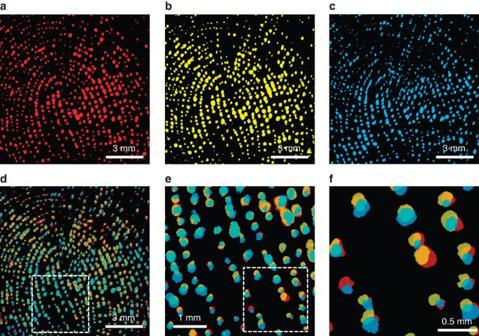Figure 6: Reliability test. (a–c) Three independently printed contrast-enhanced fluorescence microscope fingerprint images deposited by same donor. The yellow (b) and blue (c) coloured images are intentionally generated using a Photoshop programme for comparison purposes. (d) Superimposed images displayed ina–c. (e) Magnified image in the marked area ind. (f) Magnified image in the marked area ine. Figure 6: Reliability test. ( a – c ) Three independently printed contrast-enhanced fluorescence microscope fingerprint images deposited by same donor. The yellow ( b ) and blue ( c ) coloured images are intentionally generated using a Photoshop programme for comparison purposes. ( d ) Superimposed images displayed in a – c . ( e ) Magnified image in the marked area in d . ( f ) Magnified image in the marked area in e . Full size image As the hydrochromic film method enables mapping of sweat-secreting pores, it should be applicable to studies of sweat pore functions. To demonstrate this feature, five independent fingerprints from the same donor were deposited on a poly(PCDA-Cs) film in the morning, afternoon and at night during a 1-week period ( Fig. 7 ). Analysis of the resulting patterns shows that, although a majority of the sweat pores are active (dots inside the red dots in Fig. 7f ), some secrete sweat in an inconsistent manner (dots inside the triangles in Fig. 7f ) or not at all (dots inside the blue circles in Fig. 7f ) during the observation period. Thus, the hydrochromic mapping strategy enables a clear differentiation between sweat-secreting active pores and those that are inactive and, as a result, it is potentially useful for clinical diagnosis of the sweat pore function. 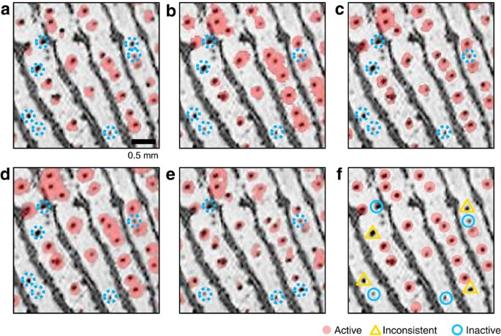Figure 7: Test of active sweat pores. (a–e) Superimposed microscope images of five independently marked fingerprints on poly(PCDA-Cs) films (pale-red-coloured dots) with digitally scanned fingertips. The black-coloured microdots are pores on the ridges. The red dot images shown ina–ewere obtained in the morning, afternoon and at night from the same donor for a 1-week period. (f) The dots inside the red circled areas are sweat-secreting active pores, while the microdots inside the blue circles are found to be inactive pores during the period of the experiment. The microdots inside the yellow triangles are partially active sweat pores. Figure 7: Test of active sweat pores. ( a – e ) Superimposed microscope images of five independently marked fingerprints on poly(PCDA-Cs) films (pale-red-coloured dots) with digitally scanned fingertips. The black-coloured microdots are pores on the ridges. The red dot images shown in a – e were obtained in the morning, afternoon and at night from the same donor for a 1-week period. ( f ) The dots inside the red circled areas are sweat-secreting active pores, while the microdots inside the blue circles are found to be inactive pores during the period of the experiment. The microdots inside the yellow triangles are partially active sweat pores. Full size image The feasibility of utilizing the sweat pore-based hydrochromic fingerprint detection system for latent fingerprint analysis was explored next. Java-based position tracking software (ImageJ) and a pore-pattern-matching programme implemented in MATLAB were used for the process (see Methods for details). The pore-pattern-matching programme was employed to compare a fluorescence image ( Fig. 8c ) and a latent fingerprint image ( Fig. 8d ), obtained by using ninhydrin staining ( Supplementary Fig. 6 ). The results, displayed as blue dots in Fig. 8c,d , show that the fingerprint patterns generated by using both methods closely match one another. This finding demonstrates that the pore-pattern-matching programme is effective. To gain further support for the reliability of the pore-matching programme, a manual comparison was also carried out. Visual inspection of an image ( Fig. 8g ), created by superimposition of the magnified boxed areas in Fig. 8c,d (displayed in Fig. 8e,f ), clearly shows that the pore-based hydrochromic sensor system is useful for fingerprint analysis (see also Supplementary Fig. 7 ). The meritorious feature of the new pore-based analysis system is further demonstrated by the observation that the fluorescence pore images match the ninhydrin-developed latent images including local sweat pores ( Supplementary Fig. 8 ). The pore-pattern-matching programme enabled correct matching of 15 out of 17 partially printed latent fingerprints with fluorescent images arising from five donors. The two incorrect matches were a consequence of the poor quality of the ninhydrin-stained latent images. Thus, if the ninhydrin-stained latent images are reasonably clear, the pore-matching programme functions with almost 100% accuracy. 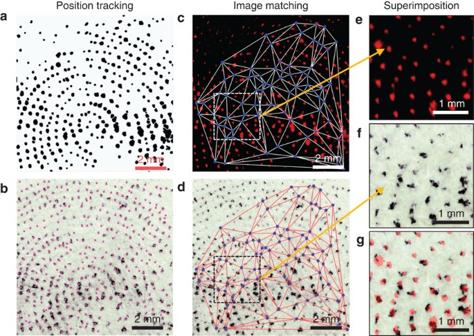Figure 8: Sweat pore-pattern matching. (a,b) Threshold images of fingerprint (a) and latent fingerprint marks (b) generated by using the position tracking method. The two images are extracted from the images shown inc,d, respectively. (c,d) A fluorescence microscopic fingerprint image printed on a hydrochromic poly(PCDA-Cs) film (c) and a latent form of the same fingerprint developed with ninhydrin (d). The blue-coloured dots, obtained using the image-matching process, indicate the matching points between the two images. (e,f) Magnified images of marked areas inc,d. (g) Superimposed image ofe,f. The latent fingerprint image shown indwas obtained by pressing a fingertip on an unmodified paper followed by staining with ninhydrin. The original purple-coloured dots obtained from ninhydrin staining were transformed to black-coloured dots using a Photoshop programme because overlapping red-coloured fluorescence images (e) with black-coloured dots (f) results in a better superimposed image (g). Figure 8: Sweat pore-pattern matching. ( a , b ) Threshold images of fingerprint ( a ) and latent fingerprint marks ( b ) generated by using the position tracking method. The two images are extracted from the images shown in c , d , respectively. ( c , d ) A fluorescence microscopic fingerprint image printed on a hydrochromic poly(PCDA-Cs) film ( c ) and a latent form of the same fingerprint developed with ninhydrin ( d ). The blue-coloured dots, obtained using the image-matching process, indicate the matching points between the two images. ( e , f ) Magnified images of marked areas in c , d . ( g ) Superimposed image of e , f . The latent fingerprint image shown in d was obtained by pressing a fingertip on an unmodified paper followed by staining with ninhydrin. The original purple-coloured dots obtained from ninhydrin staining were transformed to black-coloured dots using a Photoshop programme because overlapping red-coloured fluorescence images ( e ) with black-coloured dots ( f ) results in a better superimposed image ( g ). Full size image In order for it to be suitable for sweat pore mapping, a hydrochromic material must have several important characteristics. First, it should possess a balanced sensitivity to water in that it should be sufficiently responsive to display a colorimetric transition upon contact with the very low amounts of water secreted from sweat pores and not too sensitive so that it undergoes a colour change under ambient condition. Second, it is highly desirable that the water-promoted colorimeric transition be readily monitored using the naked eye and, therefore, that it takes place in the visible range. In addition, it would be more attractive if the hydrochromic phenomenon is accompanied by the generation (‘Turn-On’) of a colour or fluorescence upon hydration. Importantly, hydrochromic materials that display water-promoted colour or fluorescence quenching are not appropriate for sweat pore mapping because they would generate micron-sized sweat pore images that would be unrecognizable owing to the presence of dominant background signals. Finally, synthesis of the hydrochromic material and fabrication of the sensor system should be relatively simple. Fortunately, PDA-based hydrochromic sensor systems satisfy the criteria outlined above for the efficient sweat pore mapping. The colorimetric sensitivity of hydrochromic PDAs is easy to manipulate by properly choosing the diacetylene monomers and metal cations. In addition, the blue-to-red colour change as well as fluorescence ‘Turn-On’ enable the PDA-based sensor of this type to be used to monitor and image sweat-secreting active pores. Furthermore, the hydrochromic sensor film can be readily produced from commercially available diacetylene monomers. It should be noted that detection of latent fingerprint images using polymerizable diacetylenes was previously described [49] . The earlier study, however, focused on the development of latent ridge patterns. The sweat pore-mapping strategy based on the hydrochromic PDA is highly important because conventional fingerprint detection methods [39] depend heavily on friction ridge patterns and, consequently, they require large portions of a latent fingerprint for reliable analysis. In contrast, the new pore-based method can be employed for human identification even when a relatively small portion of a latent fingerprint exists. In addition, the newly developed technique to map active pores precisely should be highly useful in the clinical diagnosis of malfunctioning sweat pores. Although the experiments described above were carried out using poly(PCDA-Cs) films, the results of further studies demonstrate that PDA films derived from PCDA-Rb and TCDA-K are equally useful for fluorescence ‘Turn-On’ mapping of the active sweat pores ( Supplementary Fig. 9 ). Notably, because the poly(TCDA-K) film displays a higher stability in humid environments ( Fig. 4 ), it can be used to map sweat pores under a wide range (RH 30–90%) of humidity conditions ( Supplementary Fig. 10 ). Finally, it is believed that observation made in the current effort will open new avenues for the application of hydrochromic materials, which has been limited thus far to humidity sensing and measurement of water contents in organic solvents. General The diacetylenic lipids, PCDA, TCDA and HCDA (8,10-heneicosadiynoic acid) were purchased from GFS Chemicals, OH, USA. Film thicknesses were measured using an alpha step instrument. Contact angle data were obtained using a PHX300, Korea. Raman spectra were obtained using laser excitation at 785 nm and a Raman microscope (Kaiser Optical Systems). SEM images were obtained with a JEOL(JSM-6330F) FE-SEM, and optical/fluorescence microscopic images were collected with a Olympus BX 51W/DP70. XRD spectra were recorded with a HR-XRD, D8 discover, Bruker. Friction ridge structures on a fingertip were obtained using a video microscope system (Camscope SV 32) with a prism. A homemade humidity-controlled chamber was used for hydrochromism tests under various humidity conditions. Fabrication of a hydrochromic PDA film A typical procedure for the preparation of a hydrochromic sensor film is as follows. To an aqueous solution (0.4 ml) of cesium hydroxide (750 mg, 5 mmol) was added dropwise a tetrahydrofuran solution (9.6 ml) containing PCDA 1.87 g, 5 mmol). The resulting mixture was stirred at an ambient temperature for 1 h. The formed transparent gel was spin-coated on a PET film to make a thin film (thickness: ca. 3.8 μm). Irradiation of the monomer film with a hand-held UV lamp (254 nm, 1 mW cm −2 , 10 s) resulted in the generation of a blue-coloured hydrochromic PDA. Inkjet printing of a diacetylene suspension Ink solution (black) from a conventional inkjet office printer (HP Deskjet D2360) cartridge was removed, and the cartridge was thoroughly washed with ethanol, water and dried with N 2 blowing. A suspension (0.2 ml) containing PCDA-Cs (125 mM), prepared as described above, was loaded into the cartridge. In order to avoid cartridge clogging caused by fast solvent evaporation, the content of the organic solvent was minimized (40% v/v Dioxane-H 2 O). Printing of the diacetylene suspension on a PET film followed by UV irradiation (254 nm, 1 mW cm −2 , 10 s) afforded a flexible water-responsive colorimetric sensor film. It is more effective to add a small amount of dimethylsulphoxide to the PCDA-Cs ink medium (optimum condition, H 2 O:dioxane:THF:dimethylsulphoxide=6:4:1/20:1/40) and to filter the PCDA-Cs ink through a 0.2 μm filter to remove large aggregates. The PCDA-Cs ink prepared in this manner can be used to print more than 30 copies of clean images shown in Supplementary Movie 3 without clogging. Sweat pore mapping Fingerprinting was conducted by pressing a fingertip softly on a hydrochromic PDA film (see Supplementary Movie 5 ). Fluorescent microdots that represent the sweat-secreting active pores were analysed using a fluorescence microscope (excitation: 510–550 nm). The friction ridge patterns on a fingertip were obtained with a digital scanner equipped with a prism. An Adobe Photoshop programme was used for superimposition of the sweat pore images obtained from the hydrochromic method with the digitally scanned ridge patterns. Latent sweat pore images on paper A modified ninhydrin staining method was employed to obtain sweat pore images on a paper. A stock ninhydrin solution (1 g ninhydrin in 9 ml ethanol and 1 ml acetic acid) was diluted 20 times with methanol for a working staining solution. Fingerprinting was conducted by pressing a fingertip on an unmodified A4 paper. The diluted working ninhydrin solution was spray-coated to the fingerprinted area and the ninhydrin-treated paper was placed on a hot plate (80 °C) for 20 min for the generation of the latent fingerprint image. Sweat pore-pattern-matching process A process to match the sweat pore patterns in two images, which utilizes a Java-based image-processing tool (ImageJ) and a pore-pattern-matching programme implemented in MATLAB, was developed. The individual images are independently obtained from either a fluorescence image of a fingerprint deposited on the hydrochromic sensor or an image of a latent fingerprint obtained on paper by ninhydrin staining. To determine the sweat pore positions, the fluorescence image is thresholded to yield a binary image [50] . The coordinates of the pore positions are calculated as a centroid of each pore region in the binary image ( Fig. 8a ). For the latent fingerprint image (RGB), it is converted to greyscale with luminance defined as unweighted average of the RGB colours. The local maxima of the luminance under an appropriate value of noise tolerance ( ca. 15–25) are selected as coordinates of sweat pore positions ( Fig. 8b ). To compare two images, I and II, the pattern-matching programme implemented in MATLAB reads in the coordinates of sweat pores ( n -positions for the image-I and m -positions for the image-II). The pore-pattern-matching algorithm is composed of two stages: (1) matching target pore positions and (2) matching background pore positions. In the first stage, the distances ( d I ) between a selected pore position ( i th ) and its 15 neighbouring pores in image-I are calculated and repeated for all other pore positions ( n −1). The obtained distances ( d I ) from the i th pore are iteratively compared with those ( d II ) calculated for j th pore ( j =1, 2,…, m ) in image-II using the same procedure in order to find a sequence of minimum values of s ij =| d I − d II |. Once four or five pores in the sequence of s ij values satisfy the criterion, s ij < ε 1 =0.04 mm, the corresponding pores in both images are assigned as target pore positions. Subsequently, the relative angles ( θ I and θ II ) between the target pore positions are calculated for image-I and -II, respectively. The second criterion ( Δθ ij < ε 2 =10°) is then applied to the angle differences, Δθ ij =| θ I − θ II |, between the target positions of each image. When the second criterion is satisfied, image-II is rotated and translated so that the target positions in image-II match the corresponding positions in image-I. (If either criterion is not satisfied, the next iteration for ( i +1) th pore in image-I is executed.) In the second stage, background pore positions surrounding the target positions in the modified image-II are compared with those in image-I. Analysis of overlapping the two images identifies nearest pore positions in image-I with background pore positions in image-II. The displacements ( λ ) between the corresponding background pore positions in both images are subsequently calculated and the pore positions with the values of λ that satisfy the criterion ( λ < ε 1 ) are selected. When the number of selected pore positions is larger than a specified percentage ( ε 3 ) of the total m -positions in image-II, the two fingerprint images are assumed to match. Note that the range of ε 3 is from 8 to 30%, depending on the quality and the number of pores in image-II. How to cite this article: Lee, J. et al . Hydrochromic conjugated polymers for human sweat pore mapping. Nat. Commun. 5:3736 doi: 10.1038/ncomms4736 (2014).